Real-space observation of unbalanced charge distribution inside a perovskite-sensitized solar cell Perovskite-sensitized solar cells have reached power conversion efficiencies comparable to commercially available solar cells used for example in solar farms. In contrast to silicon solar cells, perovskite-sensitized solar cells can be made by solution processes from inexpensive materials. The power conversion efficiency of these cells depends substantially on the charge transfer at interfaces. Here we use Kelvin probe force microscopy to study the real-space cross-sectional distribution of the internal potential within high efficiency mesoscopic methylammonium lead tri-iodide solar cells. We show that the electric field is homogeneous through these devices, similar to that of a p-i-n type junction. On illumination under short-circuit conditions, holes accumulate in front of the hole-transport layer as a consequence of unbalanced charge transport in the device. After light illumination, we find that trapped charges remain inside the active device layers. Removing these traps and the unbalanced charge injection could enable further improvements in performance of perovskite-sensitized solar cells. The concept of using perovskite materials in solar cells [1] enabled the fabrication of devices with a power conversion efficiency (PCE) of >15% (refs 2 , 3 ). Devices are typically realized with a mesoporous structure consisting of an electron-extracting material such as TiO 2 filled with an electron donor material, which can also act as a light absorber. The mesoporous structure leads to more efficient light absorption and a large interface area. The interface between the light absorber and the electron or hole acceptor material facilitates the charge separation by providing an energetic offset between the conduction bands. In the case of perovskite materials, the thermal energy is sufficient to overcome the exciton binding energy, creating free charges already in the sensitizer material [4] . After charge separation it is important that charges flow selectively to the respective electrodes without significant losses due to recombination. In front of the electrodes, selective charge extraction is realized by using electron- and hole-transport materials (HTM), respectively [2] . However, efficient charge transfer into these materials depends on the charge extraction dynamics at their interfaces. It was recently shown that the light-absorbing perovskite material MAPbX 3 (here: MA=CH 3 NH 3 + and X=Cl − , I − ) has a long-range ambipolar charge transport character [5] . The remarkable properties of this perovskite material make highly efficient devices in a planar heterojunction possible (average PCE up to 12%) [6] . Furthermore, high PCE was obtained with devices based on an electrically insulating mesoporous scaffold of Al 2 O 3 instead of TiO 2 , indicating that the electron conducting properties of the TiO 2 are not required for efficient electron collection in the device [7] . To obtain more information about dynamic processes at the different internal interfaces in the various cell geometries, impedance spectroscopy was used to study lead halide perovskite-sensitized solid-state solar cells [8] , [9] . However, the analysis of impedance spectroscopy data requires complex theoretical models that neglect the interface roughness. Nevertheless, knowledge of the real-space charge distribution inside a solar cell would be beneficial. Recently, Edri et al. [10] , [11] used electron beam-induced current measurements (EBIC) to study the variations of charge separation inside the device. EBIC measurements are based on the local excitation and extraction of charge carriers by an electron beam. Experiments on a solar cell cross section showed that lead-halide-based perovskite solar cells form a p-i-n type junction and that electrons are extracted more efficiently than holes. However, EBIC measurements do not represent a solar cell under typically working conditions, that is, a homogeneous illumination with a broadband light source. Furthermore, measurements representing dark conditions cannot be performed. Thus, electrical potentials at interfaces and the electric field distribution inside organo-lead-halide-based solar cells remain speculative. Kelvin probe force microscopy (KPFM), an electrical operation mode of scanning force microscopy (SFM), has emerged as a powerful method to study solar cell devices [12] as it allows the simultaneous mapping of the topography and the local contact potential difference (CPD) between tip and sample with nanometer resolution. In particular, it has previously been used to study the electrical potential distribution across the internal interfaces of inorganic solar cell devices [13] , [14] , [15] . Recently, cross sections of organic bulk heterojunction solar cells made of poly(3-hexylthiophene):1-(3-methoxycarbonyl)propyl-1-phenyl[6,6]C61 (P3HT:PCBM) have been studied intensively [16] , [17] , [18] , [19] . Here, we study a highly efficient mesoscopic lead methylammonium tri-iodide solar cell based on the concept reported by Burschka et al. [2] Cross sections were polished by means of focused ion beam (FIB) such that the full structure and functionality of the device were preserved. This way, the internal interfaces between the different materials in the cell are accessible for KPFM. We mapped the CPD distribution across the active layers and correlated the measured potentials with the positions of material interfaces in the device. On illumination and under short-circuit conditions, the sample exhibited an accumulation of holes in the perovskite-rich capping layer on top of the mesoporous structure. This accumulation indicates a reduced hole extraction into the HTM compared with the electron extraction into the TiO 2 . This conclusion is supported by experiments on identically prepared devices without HTM. Here, no accumulation of holes in front of the Au electrode was observed. Consequently, the measured CPD increase in front of the HTM can be attributed to a limitation of charge extraction given by the bulk material properties. A comparison of the electrical potential distributions before and after illumination of the device revealed a persistent positive charging in the mesoporous TiO 2 and negative charging inside the perovskite capping layer, respectively. Characterization We have prepared a lead halide perovskite (CH 3 NH 3 PbI 3 ) solar cell with a 300-nm-thick mesoporous TiO 2 scaffold. This solar cell showed an open-circuit potential of V oc =0.97 V, a short-circuit current density of J sc =19.05 mA cm −2 and a fill factor of 0.66 ( Fig. 2a ). This yields a PCE of 12.54%, which is comparable to the PCEs of the state-of-the-art devices published so far. To perform cross-sectional KPFM on a working solar cell, the device was cleaved directly after preparation and the cross section was polished by FIB (details provided in Methods). We compared the J-V characteristics of an untreated reference with a FIB-polished sample after every preparation step to rule out preparation induced artifacts in the device ( Supplementary Fig. 1a ). These measurements showed that there is no relevant influence of the FIB preparation on the PCE. The major loss in PCE arises from the degradation of materials with time. After the polishing process, the device was mounted in a sample holder that allows simultaneous investigation by SFM and illumination by white light through the glass substrate ( Fig. 1 ). Contacts on the sample holder allowed us to connect the two electrodes electrically. In this way, we were able to realize different working conditions of a solar cell, namely open- and short-circuit conditions, while studying the electrical potential distribution in the solar cell. After the SFM investigation, we recorded the photoelectrical characteristics again ( Supplementary Fig. 1b ). The solar cell still exhibited the same V oc but a reduced J sc value, indicating functionality of the device during the SFM study. Figure 2: Electrical and cross-sectional characterization of the device. 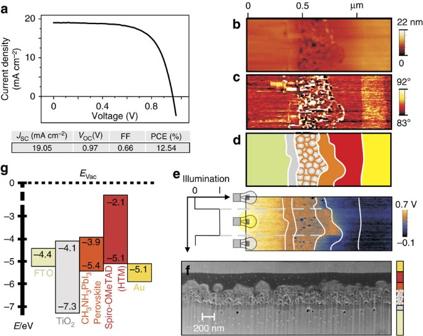Figure 2: Electrical and cross-sectional characterization of the device. (a) Current density-voltage (J-V) curve and device parameters of the sample. (b) AFM topography and (c) phase contrast images of the FIB-polished area. Within the mesoporous layer, we measured a root mean square surface roughness of 2.6 nm, indicating partially empty pores. Peak-to-peak heights correspond to thez-scale of the image. (d) Based on both images, we were able to define the material interfaces of the perovskite solar cell (white lines). (e) KPFM CPD map of the same area shown inbandcrecorded under short-circuit conditions. For clarity, we have indicated interfaces with white lines. During KPFM mapping, the illumination of the solar cell was switched on (centre). (f) SEM micrograph of a FIB polished area. The perovskite capping layer varies in thickness from 0 to 200 nm. Furthermore, perovskite crystals were observed on top of the mesoporous TiO2layer. The SEM image was recorded at a different position of the sample than KPFM to avoid SEM induced contaminations. (g) Energy level diagram of the device layer structure. ( a ) Current density-voltage (J-V) curve and device parameters of the sample. ( b ) AFM topography and ( c ) phase contrast images of the FIB-polished area. Within the mesoporous layer, we measured a root mean square surface roughness of 2.6 nm, indicating partially empty pores. Peak-to-peak heights correspond to the z -scale of the image. ( d ) Based on both images, we were able to define the material interfaces of the perovskite solar cell (white lines). ( e ) KPFM CPD map of the same area shown in b and c recorded under short-circuit conditions. For clarity, we have indicated interfaces with white lines. During KPFM mapping, the illumination of the solar cell was switched on (centre). ( f ) SEM micrograph of a FIB polished area. The perovskite capping layer varies in thickness from 0 to 200 nm. Furthermore, perovskite crystals were observed on top of the mesoporous TiO 2 layer. The SEM image was recorded at a different position of the sample than KPFM to avoid SEM induced contaminations. 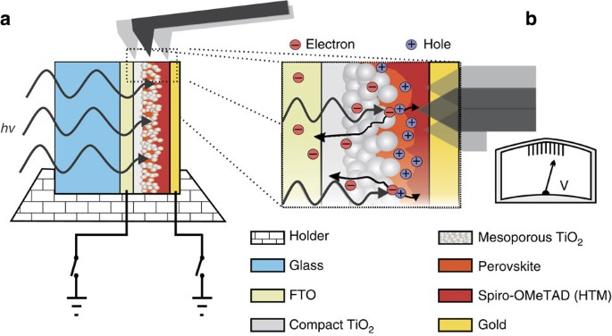( g ) Energy level diagram of the device layer structure. Figure 1: Setup of the SFM measurement principle. (a) Side view of the measurement principle. The CPD can be measured in dark and under illumination. Furthermore, the Au and fluorine-doped tin oxide (FTO) electrode can be disconnected or grounded to realize different working conditions of the device. By using SFM and KPFM, we obtain a real-space image of material interfaces (roughness and material contrast), material work functions and local charge-carrier accumulation on illumination. (b) Zoom-in and top view sketch of the material interfaces as seen by SFM in a FIB-polished area. Full size image Figure 1: Setup of the SFM measurement principle. ( a ) Side view of the measurement principle. The CPD can be measured in dark and under illumination. Furthermore, the Au and fluorine-doped tin oxide (FTO) electrode can be disconnected or grounded to realize different working conditions of the device. By using SFM and KPFM, we obtain a real-space image of material interfaces (roughness and material contrast), material work functions and local charge-carrier accumulation on illumination. ( b ) Zoom-in and top view sketch of the material interfaces as seen by SFM in a FIB-polished area. Full size image The analysis of the FIB-polished area with SFM revealed a root mean square surface roughness <3.4 nm on an area of 2.5 μm 2 ( Fig. 2b ). The granular morphology of the nominally 300 to 350-nm-thick mesoporous TiO 2 can be clearly observed at the centre of the image, assembled on top of the 80-nm-thick compact TiO 2 layer and the FTO electrode. Towards the right side, a capping layer follows consisting of bulk perovskite with a thickness ranging from 0 to 200 nm. This layer is followed by the 150 to 300-nm-thick HTM 2,2′,7,7′-tetrakis( N , N -di- p -methoxyphenylamine)-9,9′-spirobifluorene (Spiro-OMeTAD) and the Au electrode. In combination with the simultaneously captured SFM phase image ( Fig. 2c ), the interfaces between the different layers were identified and traced with white lines ( Fig. 2d ). We transferred these interface lines directly into the simultaneously recorded CPD map ( Fig. 2e ). Most of the internal interfaces appear as straight lines in the cross section, indicating sharp and well-defined interfaces between the materials. Only the interfaces between the mesoporous TiO 2 and the perovskite capping layer and between the perovskite and the HTM are rough [20] . The layers and their characteristic interface structure were also observed by complementary scanning electron microscopy studies (SEM, Fig. 2f ). Neither SFM nor SEM revealed any signs of delamination of layers at their respective interfaces during the preparation of the cross section. Thus, the material interfaces were mechanically intact, which indicates firm electrical contact between the layers. Short-circuit conditions before illumination First, we selected an area having a ≈200 nm thick perovskite capping layer ( Fig. 3a ). KPFM measures the CPD and is thus sensitive to the surface work functions Φ of the materials. Assuming that the tip work function remains constant during a line scan, the CPD reflects the built-in potential of the device. We found a decreasing CPD from the FTO (0.6 V) towards the Au electrode (≈0 V, black line profile in Fig. 3b,c ). The difference between these two values corresponds to the differences of the work function of FTO ( Φ FTO /e ≈4.4 V) (ref. 21 ) and Au ( Φ Au /e ≈5.1 V) (ref. 22 ) as sketched in the energy level diagram ( Fig. 2g ) [23] . Therefore, we conclude that the FIB-polished surfaces on the cross section are not contaminated, for example, by implanted Ga + ions. This conclusion is supported by energy dispersive X-ray spectroscopy (EDX) analysis of the as-prepared interface ( Supplementary Fig. 2 ). Furthermore, adsorbed water on the surface may have altered the absolute value of the CPD, but not the relative difference between the studied materials. The monotonically decreasing CPD from the FTO towards the Au electrode indicates the presence of a homogeneous electric field throughout the device ( E~− dCPD/d x ). A constant electric field distribution is consistent with a p-i-n type solar cell where the intrinsic material is the perovskite [24] . In particular, our measurement did not reveal a significant electrical potential drop at the interface between the perovskite layer and the HTM as suggested by Edri et al. [11] An electrical potential drop at that interface would decrease the electric field magnitude in the light absorbing perovskite layers and thus would be unfavourable. 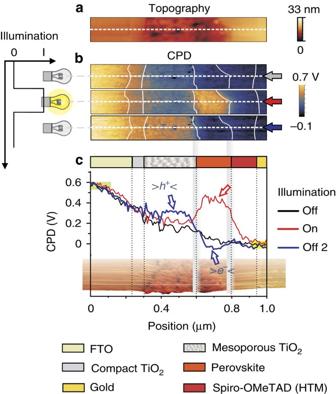Figure 3: KPFM results for short-circuit conditions. (a) Topography image of the device with a ≈200 nm thick perovskite capping layer (b) Corresponding CPD maps and (c) line profiles for short-circuit conditions before illumination (black line), during illumination (red line) and immediately after illumination (blue line). The increase in potential after turning on the illumination corresponds to an accumulation of holes inside the capping layer (red arrow). After switching off the light, trapped holes become visible inside the mesoporous structure with an increase in potential (>h+<) and trapped electrons become visible in the perovskite capping layer (>e–<). Figure 3: KPFM results for short-circuit conditions. ( a ) Topography image of the device with a ≈200 nm thick perovskite capping layer ( b ) Corresponding CPD maps and ( c ) line profiles for short-circuit conditions before illumination (black line), during illumination (red line) and immediately after illumination (blue line). The increase in potential after turning on the illumination corresponds to an accumulation of holes inside the capping layer (red arrow). After switching off the light, trapped holes become visible inside the mesoporous structure with an increase in potential (> h + <) and trapped electrons become visible in the perovskite capping layer (> e – <). Full size image Short-circuit conditions on illumination On illumination, free charge carriers are generated in the active layers of the device. A crucial parameter for a high J sc is the charge-carrier extraction across the internal interfaces. In particular, interfaces between organic and inorganic materials are delicate because the charge transport properties are usually very different. Different charge-carrier mobilities in different materials or inefficient charge extraction between adjacent layers can lead to the accumulation of charges in the cell. To study such charging effects, we kept the device under short-circuit conditions while illuminating the sample ( Fig. 3c —red line profile). Under these conditions, we measured an increase in CPD of up to 0.4 V in the perovskite capping layer, which almost reached the CPD of the FTO. This increase in CPD corresponds to the presence of additional positive charge carriers and indicates that the extraction of electrons via the TiO 2 is more efficient than the extraction of holes via the HTM. Thus, the charge transport is unbalanced in the device. The accumulation of holes prevents an efficient charge transport to the respective electrodes and thereby reduces the short-circuit current of the device. The measured CPD distribution also allows insights into the location of the charge-carrier generation process. If the charges were generated in the mesoporous layer only, we would expect a constant distribution of the CPD throughout the mesoporous and the perovskite capping layer owing to a pile-up of charges towards the HTM. Surprisingly, we observed only a small increase in CPD inside the mesoporous TiO 2 /perovskite layer. Considering the strong local light-induced increase of the CPD on the perovskite capping layer, we suggest that a significant part of charge-carrier generation takes place here. This suggestion is supported by the analysis of positions with different capping layer thickness in the solar cell ( Fig. 4a,b ). On positions with a locally thinner capping layer, the maximum in CPD inside this layer decreased (thickness 140 nm) and completely disappeared at places with a very thin capping layer (thickness 70 nm). 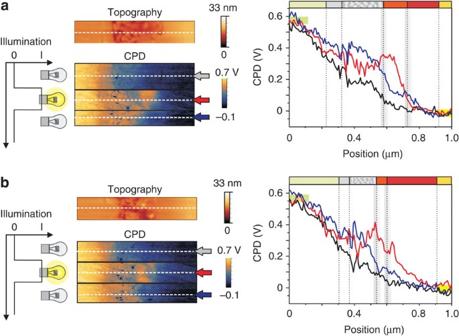Figure 4: KPFM measurements for short-circuit conditions at thinner capping layer thicknesses. (a) The CPD line profiles recorded at a capping layer thickness of ≈140 nm showed a decreased light-induced charging in the capping layer compared with the 200-nm thick one. (b) CPD line profiles at an area where the perovskite capping layer was ≈70 nm. Here, the CPD reached a maximum at the mesoporous–perovskite capping layer interface. Figure 4: KPFM measurements for short-circuit conditions at thinner capping layer thicknesses. ( a ) The CPD line profiles recorded at a capping layer thickness of ≈140 nm showed a decreased light-induced charging in the capping layer compared with the 200-nm thick one. ( b ) CPD line profiles at an area where the perovskite capping layer was ≈70 nm. Here, the CPD reached a maximum at the mesoporous–perovskite capping layer interface. Full size image Short-circuit conditions after illumination Directly after the illumination, the CPD distribution did not completely return to the initial level ( Fig. 3c —blue line profile). For positions with a thick capping layer, the CPD in the mesoporous TiO 2 layer increased to values higher than in the illuminated case. At the same time, the CPD value inside the capping layer decreased below the initial CPD before illumination. In other words, the mesoporous layer contained excess holes (> h + < in Fig. 3c ) and the perovskite layer contained excess electrons (> e − < in Fig. 3c ). Both types of charge carriers are no longer mobile, at least not within the time scale of the experiment (10 min). Thus, these charge carriers could have been trapped by defects in the material. Those trapped charges could contribute to hysteresis in J–V curves as reported by Snaith et al. [25] Interestingly, we found that the measured CPD on the mesoporous and perovskite capping layer after illumination depends on the thickness of the perovskite capping layer ( Fig. 4a,b ). For areas with a locally thinner capping layer, the number of trapped holes is reduced and trapped electrons are not visible any more. This may be a consequence of a different defect density or depth of traps. Charges in the electric field In the following, we want to discuss the impact of the observed charge distributions on the device physics, which were observed on and after illumination. First, we propose a model that elucidates the consequence of the electrical potential barrier in front of the HTM. We take a closer look at the electric field distribution in the illuminated case, that is, the derivative of the CPD with respect to the cross-sectional coordinate (−dCPD/d x, Fig. 5 ). The strong accumulation of holes in the perovskite capping layer during the illumination produces an electric field that repels holes from this layer. On one hand, holes within the perovskite capping layer will be driven to the HTM (right side, positive electric field), where they can be extracted to the Au electrode. On the other hand, it is energetically unfavourable for holes generated in the mesoporous layer to overcome this electrical potential barrier and reach the electrode. In addition, some of the holes in the perovskite capping layer are even driven towards the mesoporous layer (left side, negative electric field), where they either recombine or become trapped. Therefore, we conclude that the electrical potential barrier reduces the short-circuit current. Second, the KPFM measurement under illumination represents a dynamic equilibrium between continuous charge generation, charge extraction and recombination at interfaces and traps. So traps in the materials are filled with the respective charge carriers on illumination. Trapped holes are not visible in the mesoporous layer by KPFM as they are screened by adjacent, photogenerated electrons. Now, when the illumination is switched off, trapped holes remain and a higher CPD is measured (> h + < in Fig. 3a ). A similar scenario is also feasible for the measured additional electrons in the perovskite capping layer after illumination (> e − < in Fig. 3a ). Here, the energy level diagram ( Fig. 2g ) suggests that it is unfavourable for electrons to move from the TiO 2 into the perovskite capping layer. Thus, the measured decrease in CPD is due to trapped electrons that are already present during the illumination. Finally, it should be mentioned that these conclusions originate from our observations during the KPFM measurements and need to be verified by other techniques and theoretical device modelling. 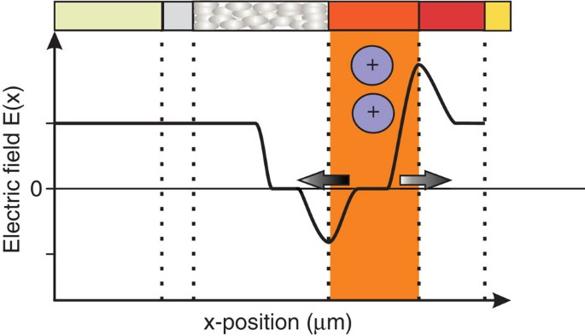Figure 5: Schematic outline of the field distribution inside the device on illumination. The electric field is determined from CPD measurements (E(x)=−dCPD/dx) under illumination (see alsoFig. 3c). Figure 5: Schematic outline of the field distribution inside the device on illumination. The electric field is determined from CPD measurements ( E(x) =−dCPD/d x ) under illumination (see also Fig. 3c ). Full size image Measurement without hole transporting material Principally, surface defects could also be generated by the FIB polishing step during sample preparation. To exclude such surface defects and band bending due to the applied KPFM voltages as the origin on the accumulation of charges in the perovskite capping layer, we prepared a state-of-the-art device (PCE 5.6%) without HTM as a reference. The lower efficiency of such a device is a consequence of the recombination of electrons in the perovskite with holes at the Au electrode interface. In this case, accumulation of holes according to our proposed unbalanced charge extraction mechanism should not occur in the perovskite capping layer owing to the ohmic contact with the Au electrode. Under short circuit conditions and in dark, the CPD measurements revealed a difference of ~0.5 V in CPD between the FTO and the Au electrode material ( Fig. 6 —black line profile). This value is consistent with the CPD difference in the previous measurement of the sample with HTM ( Fig. 3 ). On illumination, the CPD did not change significantly and thus no charging of layers occurred ( Fig. 6 —red line profile). Consequently, we can exclude secondary effects from the sample preparation and the KPFM experimental procedure as the reason for the observed light-induced CPD increase in front of the HTM. 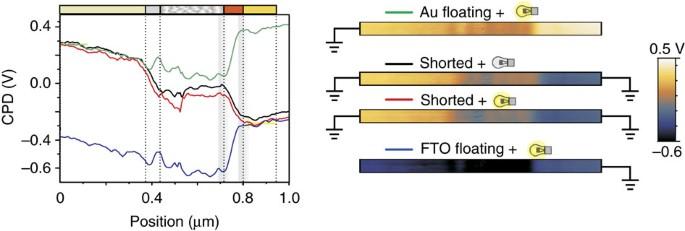Figure 6: CPD measurements of the device without HTM. The black line is the CPD profile for short-circuit conditions (shorted) in dark. On illumination (red line profile), no significant increase in CPD was measured in the perovskite capping layer (marked in orange on top of the graph). The CPD distribution for open-circuit conditions showed that the examined area was functional, that is, positive charging of the Au cathode (green line) and negative charging of the FTO anode (blue line) as expected from the device J-V curves. Figure 6: CPD measurements of the device without HTM. The black line is the CPD profile for short-circuit conditions (shorted) in dark. On illumination (red line profile), no significant increase in CPD was measured in the perovskite capping layer (marked in orange on top of the graph). The CPD distribution for open-circuit conditions showed that the examined area was functional, that is, positive charging of the Au cathode (green line) and negative charging of the FTO anode (blue line) as expected from the device J-V curves. Full size image Open-circuit conditions on illumination To study the electrical potential distribution under open-circuit conditions, we disconnected one electrode (floating potential) but kept the other one grounded ( Fig. 7a,b ). Both measurements revealed that the electrodes charge up to a ΔCPD of ±0.8 V, respectively. This value is very close to the measured open-circuit potential of the device measured with a voltmeter (0.97 V) on contacts coming out from the sample holder. Furthermore, it is in good agreement with a measurement of the ΔCPD on top of the HTM of a similar solar cell in the dark and on illumination [23] . In both cases (Au and FTO floating), the CPD is not constant within the perovskite capping layer, whereas it is nearly constant in all other layers. By comparing the CPD characteristics under short-circuit and open-circuit conditions ( Fig. 7a ), it becomes evident that the open-circuit potential builds up mainly in the perovskite capping layer. This observation further supports our earlier conclusion that an important part of the charge-carrier generation and separation takes place in that layer. 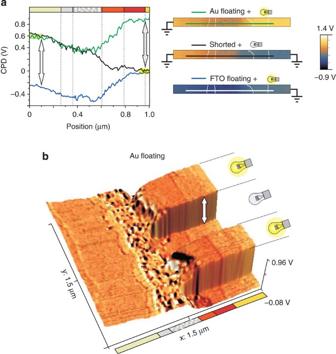Figure 7: KPFM results for open-circuit conditions. (a) CPD line profiles for open-circuit conditions on illumination compared with dark short-circuit conditions. Both arrows indicate the charging of the respective electrodes, ΔCPD~800 mV. The dotted lines correspond to the interfaces of the solar cell. (b) Three-dimensional (3D) visualization of electrical potential change for open-circuit conditions with Au electrode floating. The magnitude of the CPD is plotted in 3D to visualize changes on illumination within the perovskite capping layer. The colour overlay corresponds to the topography. Here, illumination was switched on and off two times and ΔCPD is indicated by an arrow. Figure 7: KPFM results for open-circuit conditions. ( a ) CPD line profiles for open-circuit conditions on illumination compared with dark short-circuit conditions. Both arrows indicate the charging of the respective electrodes, ΔCPD~800 mV. The dotted lines correspond to the interfaces of the solar cell. ( b ) Three-dimensional (3D) visualization of electrical potential change for open-circuit conditions with Au electrode floating. The magnitude of the CPD is plotted in 3D to visualize changes on illumination within the perovskite capping layer. The colour overlay corresponds to the topography. Here, illumination was switched on and off two times and ΔCPD is indicated by an arrow. Full size image Performing similar experiments on the device without HTM also resulted in a charge up of the electrodes ( Fig. 6 , green and blue line). For a floating Au electrode, it charged up by a ΔCPD of ~0.6 V. Furthermore, the CPD potential drops inside the perovskite capping layer but stays above the CPD values measured for short-circuit conditions. Then at the position of the compact TiO 2 layer, the CPD overlaps with the ones measured under short-circuit conditions. This positive offset can be attributed to more holes in the mesoporous and perovskite capping layer for open circuit conditions. Only at the interface with the compact TiO 2 these holes can recombine with electrons. Such an offset was not observed for a device that was made with a HTM. So the role of the HTM is unquestionable for achieving selective charge transfer as expected by the energy level diagram. Elemental analysis To verify the elemental composition in the device and thus its functional components, we performed scanning transmission electron microscopy (STEM) in combination with EDX on cross sections of these devices ( Fig. 8 ). For this purpose, a thin lamella of the solar cell was prepared by FIB and subsequently transferred to a TEM grid. The elemental analysis showed that the Ti distribution is in agreement with the suggested cell structure: a bulk TiO 2 layer on top of FTO, followed by a mesoporous layer. This mesoporous layer contains Ti at a lower concentration than the compact layer. Furthermore, STEM–EDX showed that Pb is present throughout the mesoporous layer with a homogenous distribution. The highest Pb concentration corresponds to the perovskite capping layer. In this layer, we recorded no signal from Ti and C. To mention here, the structure of the capping layer is consistent with SFM and SEM ( Fig. 2b,c,f ). 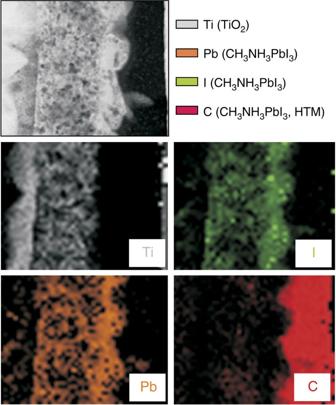Figure 8: Cross-sectional elemental analysis. STEM micrograph and corresponding elemental maps showing the relative distribution of Ti, Pb, I and C. Figure 8: Cross-sectional elemental analysis. STEM micrograph and corresponding elemental maps showing the relative distribution of Ti, Pb, I and C. Full size image We show for the first time a real-space analysis of the photoinduced changes in the internal electrical potentials of a highly efficient lead halide perovskite solar cell. KPFM gave insight into the internal electrical potential distribution across the functional layers of a solar cell device. From these electrical potential distributions, we derived the electric field distribution in the solar cell resembling a p-i-n type junction. In particular, we observed an unbalanced charge-carrier extraction from the perovskite-rich capping layer under short-circuit conditions, which is consistent with EBIC data [11] . The consequent accumulation of excess holes in this layer creates an electrical potential barrier that reduces the short-circuit current. This electrical potential barrier may be one bottleneck for improving the efficiency of the standard mesoscopic perovskite based solar cell systems. To overcome this bottleneck, new materials for the HTM might lead to a more balanced charge extraction and will push the light-harvesting abilities. The KPFM method allows us not only to map the local CPD response but also to correlate it with the local structure of the functional layers. We concluded that free charge carriers are also generated inside the perovskite layer by comparing the CPD response at different positions with the perovskite capping layers of different thicknesses. The hysteresis in the CPD on illumination and subsequent dark measurements indicated the presence of traps in the mesoporous layer. Knowledge of the electric field distribution in mesoscopic solar cell devices and the position of trapped charges will allow a further estimation of the energy of trapped charges. Materials The chemicals and solvents were either purchased from Sigma Aldrich or Agros and were employed without any further treatment or purification. 18NR-T paste from Dyesol was employed for mesoporous TiO 2 film fabrication. 2,2′,7,7′-tetrakis( N , N -di- p -methoxyphenylamine)-9,9′-spirobifluorene (Spiro-OMeTAD) was purchased from Merck KGaA. Methylammonium iodide, CH 3 NH 3 I (MAI), was synthesized in accordance with the literature [26] . Device fabrication FTO-coated, 3-mm-thick glass (NSG10) was patterned by laser etching. Then, the substrates were cleaned and brushed using Hellmanex solution and rinsed with deionized water and ethanol; subsequently, they were ultrasonicated in 2-propanol and rinsed again with ethanol and finally dried with compressed air. Before the compact layer deposition, the samples were cleaned with an ultraviolet/O 3 treatment for 30 min. The TiO 2 compact layer was deposited by spin coating an aqueous TiCl 4 solution (2 M) at 5,000 r.p.m. for 30 s. Then, the samples were heated at 125 °C for 30 min. The TiO 2 mesoporous layer was prepared by spreading a solution of the commercial 18NR-T paste of Dyesol diluted in pure ethanol (1 g of paste in 3.5 g of ethanol) over the compact titania layer, and spin coated at 5,000 r.p.m. for 30 s. Then, the samples were sequentially heated to 125 °C (5 min), 325 °C (5 min), 375 °C (5 min), 450 °C (15 min) and finally 500 °C (15 min) for the sintering process. Next, the perovskite was prepared by sequential deposition [2] . For this, a first lead iodide (PbI 2 ) film was deposited by spin coating (6,500 r.p.m. for 30 s with 5,500 r.p.m. s −1 as acceleration) using 50 μl per cell of PbI 2 solution in N , N -dimethylformamide that was kept at 70 °C under vigorous stirring. Immediately after the spin-coating step, the cells were placed onto a hot plate at 70 °C for 30 min for annealing. The samples were allowed to cool to room temperature, after which the cells were dipped in the MAI solution in 2-propanol (8 mg ml −1 ) for 20 s until the change of colour from yellow to dark brown–black was observed. Subsequently, they were rinsed in pure 2-propanol and dried using the spin-coating machine at 4,000 r.p.m. for 30 s. Then, the samples were annealed again at 70 °C for 30 min. For hole transporting materials, 35 μl of the Spiro-OMeTAD solution was spin coated at 4,000 r.p.m. for 30 s. The Spiro-OMeTAD solution was made by dissolving 72.3 mg of Spiro-OMeTAD in 1 ml of chlorobenzene; 21.9 μl of tris (2-(1H-pyrazol-1-yl)-4-tert-butylpyrydine)cobalt(III) bis(trifluoromethylsulphonyl)imide (FK209) stock solution (400 mg of FK209 in 1 ml of acetonitrile), 17.5 μl of lithium bis(trifluoromethylsulphonyl)imide (LiTFSI) stock solution (520 mg of LiTFSI in 1 ml of acetonitrile) and 28.8 μl of 4-tert-butylpyridine (tBP) were also added to the solution as additives. The cells were finally completed by thermally evaporating 150 nm of gold as a cathode under a vacuum level between 1 × 10 −6 and 1 × 10 −5 torr. PbI 2 , MAI and Spiro-OMeTAD solutions were prepared inside an argon glove box under moisture and oxygen-controlled conditions (H 2 O level: <1 p.p.m. and O 2 level: <50 p.p.m.). PbI 2 spin-coating, MAI dipping and Spiro-OMeTAD spin-coating depositions were developed inside a dry box. The reference sample without Spiro-OMeTAD was fabricated in the same procedure, but PbI 2 was employed as 1.25 M instead of 1 M and no further HTM was deposited on these devices. Device characterization For the current density versus voltage analysis before preparation, we used a setup consisting of a 450 W Xe lamp (Oriel) with a Schott K113 Tempax sunlight filter (Praezisions Glas & Optik) as a light source. A digital source meter (Keithley Model 2400) was used to apply the voltage to the cell while the current was recorded. The active area was fixed at 0.2025, cm 2 using a metal mask. For the J–V curve after the measurements, a 150 W Xe lamp (Oriel) with a UVB/UVA dichroic mirror (280 – 400 nm) was employed as the light source. A digital source meter (Keithley Model 2400) was used to apply the voltage to the cell while the current was recorded. The active area was 0.24 cm 2 . Device preparation for KPFM With a dual-beam FIB (FEI Nova600 Nanolab), we deposited a 2-μm-thick Pt protection layer measuring 50 × 5 μm on the top electrode. This Pt bar was placed 5 μm below the broken edge to eliminate contamination and therefore short cuts of the deposited Pt with the cleaved surface. For the following polishing steps, the ion beam was positioned parallel to the cross section perpendicular to the Pt bar. This geometry was used to reduce the contamination with Ga ions of the Gaussian shaped beam and the layer system (TEM and Sup. EDX). Thereby, the Pt bar acted as a shield and protected the layers from the Ga ions beside the focused position. The polishing of the cross section was then done in two steps. First, a coarse polishing step was performed at an acceleration voltage of 30 kV and a current of 3 nA for a volume of 60 × 5 × 10 μm 3 . Later, a fine polishing step created a smooth surface with an acceleration voltage of 30 kV and a current of 100 pA for a volume of 30 × 1 × 5 μm 3 . Particularly, the second polishing step directly milled at the Pt-protected area. After the FIB preparation, the sample was transferred in air to the SFM setup with a transfer time of less than 10 min. KPFM To avoid cell degradation, for example, by photo-oxidation or humidity [27] , an Asylum Research MFP3d scanning force microscope was operated in a glove box filled with dry nitrogen. We used a PPP-EFM cantilever at a resonance frequency of 68.587 kHz and an oscillation amplitude of ~70 nm. Double sideband frequency modulation KPFM [28] , [29] was done with the topographic and electrical potential feedback set over an external Zurich Instruments HF2LI-MOD lock-in amplifier at a modulation frequency of 1 kHz and an a.c. tip voltage of 3 V in single scan mode. The feedback d.c. potential was applied to the tip, thus e × V CPD = Φ tip — Φ sample . We chose a scan rate of 0.6 Hz. The sample was fixed in a custom-made vertical sample holder with electrical connections to both of the electrodes. These connections were accessible from outside the glove box. For short-circuit conditions, both electrodes were put on the same ground electrical potential as the lock-in amplifier. Open-circuit conditions were simulated by disconnecting one electrode. We illuminated the device with a UVICO-VIS broadband white light source (spectra see http://www.rapp-opto.com/continuous-light-sources.html ) with an intensity of ~1,000 W m −2 focused on the sample and filtered through an additional band pass filter (Schott KG 3 transmission >50% from 350 to 700 nm) to reduce the heating of the device and thereby the drift during the measurement. Bright-field mode TEM and energy-filtered TEM Electrospray ionization measurements: For the cross-sectional analysis by TEM, a lamella was prepared by a dual-beam FIB (FEI Nova600 Nanolab) from the perovskite solar cell. To shield the sample from implantation of the Ga + ions, a 200-nm-thick Pt layer was deposited initially with the electron beam at 5 kV, 1.6 nA. Subsequently, Pt was deposited on the same area using the ion beam until the desired thickness of approx. 2 μm was reached. Then the AUTO TEM software was used to cut the two trenches from both sides at 30 kV and 0.3 nA. The thickness of the lamella was about 1 μm. During the lift-out step, the Omnipobe micromanipulator (thin tungsten needle) was approached into contact with the lamella. Then the Omniprobe was glued to the lamella by depositing a small Pt spot. Afterwards, the lamella was transferred to the TEM copper grid holder with the Omniprobe micromanipulator, where it was fixed again by depositing a small Pt spot. After separation of the lamella by FIB, it was thinned and polished at a decreasing ion current ranging from 0.3 nA to 30 pA at 30 kV in three steps from both sides. The final thickness of the lamella was approximately 100 nm. The TEM measurements were performed using an acceleration voltage of 200 kV on a Tecnai F20 (FEI) transmission electron microscope equipped with an energy dispersive X-ray spectrometer (EDAX). STEM in combination with EDX provides precise elemental maps by means of locally recording the spectrum of emitted X-rays. It should be noted that the resulting elemental maps yield only a relative concentration distribution. SEM measurements: For SEM measurements, we used the same samples as those prepared for KPFM. Measurements were conducted with a Zeiss 1530 Gemini scanning electron microscope using a landing energy of the probe electrons of 1 keV. For compositional elemental information, we used a Hitachi SU 8000 SEM equipped with a Bruker XFlash silicon drift detector for X-ray spectroscopy microanalysis. To achieve sufficient X-ray excitation, we operated the SEM at an acceleration voltage of 10 kV using analytical working conditions. How to cite this article: Bergmann, V. W. et al. Real-space observation of unbalanced charge distribution inside a perovskite-sensitized solar cell. Nat. Commun. 5:5001 doi: 10.1038/ncomms6001 (2014).